Coordinated activation of the Rac-GAP β2-chimaerin by an atypical proline-rich domain and diacylglycerol Chimaerins, a family of GTPase activating proteins for the small G-protein Rac, have been implicated in development, neuritogenesis and cancer. These Rac-GTPase activating proteins are regulated by the lipid second messenger diacylglycerol generated by tyrosine kinases such as the epidermal growth factor receptor. Here we identify an atypical proline-rich motif in chimaerins that binds to the adaptor protein Nck1. Unlike most Nck1 partners, chimaerins bind to the third SH3 domain of Nck1. This association is mediated by electrostatic interactions of basic residues within the Pro-rich motif with acidic clusters in the SH3 domain. Epidermal growth factor promotes the binding of β2-chimaerin to Nck1 in the cell periphery in a diacylglycerol-dependent manner. Moreover, β2-chimaerin translocation to the plasma membrane and its peripheral association with Rac1 requires Nck1. Our studies underscore a coordinated mechanism for β2-chimaerin activation that involves lipid interactions via the C1 domain and protein–protein interactions via the N-terminal proline-rich region. Chimaerins represent a class of GTPase activating proteins (GAPs) for the small G-protein Rac that have been implicated in development, axon guidance, metabolism, cell migration and T-cell activation [1] , [2] , [3] , [4] , [5] , [6] , [7] . Chimaerin family members (α1-, α2-, β1- and β2-chimaerin) act as effectors of tyrosine kinases such as epidermal growth factor receptor (EGFR) or Eph receptors and G-protein coupled receptors [2] , [6] , [8] , [9] . Deregulation of CHN genes has been recently associated with human pathologies including autosomal dominant Duane retraction syndrome, schizophrenia, insulin resistance, intrauterine growth deficiency, ischaemic stroke and cancer [4] , [10] , [11] , [12] , [13] , [14] . The molecular basis for the regulation of chimaerin Rac-GAPs remains poorly understood. At a structural level chimaerins have a conserved GAP domain responsible for the acceleration of GTP hydrolysis by Rac and a C1 domain with high homology to the phorbol ester-binding site in protein kinase C (PKC). A unique feature of chimaerin Rac-GAPs is that they are regulated by diacylglycerol (DAG), a lipid second messenger generated by phospholipase C (PLC) in response to both G-protein coupled receptor and tyrosine kinase receptor activation [15] . DAG (or phorbol ester) binding to the C1 domain represents an essential step for anchoring chimaerins to the plasma membrane, where they associate with active Rac (Rac-GTP) to promote its inactivation [9] . In analogy with PKCs, DAG binding to the C1 domain in chimaerins requires acidic phospholipids in the inner layer of the plasma membrane, primarily phosphatidylserine (PS) [16] , [17] . α2- and β2-chimaerins, spliced variants of CHN1 and CHN2 genes, respectively, have an SH2 domain in the N-terminal region [18] , [19] . They are autoinhibited by intramolecular interactions between the C1 domain and other regions including the SH2 domain, the GAP domain, and the SH2-C1 linker. The C1 domain is buried within the structure and, therefore, binding of DAG or DAG-mimetics is insufficient to promote the translocation of α2- and β2-chimaerins to membranes, unless high ligand concentrations are used [5] , [20] . On the other hand, full translocation is observed in response to physiological stimuli capable of generating DAG, such as epidermal growth factor (EGF) [5] , [9] . Thus, lipid binding to the C1 domain is not sufficient for chimaerin translocation, and other mechanisms triggered by tyrosine kinase receptor activation must be required for protein anchoring to membranes. Chimaerins physically and functionally interact with Nck1 and Nck2, adaptor proteins originally identified as regulators of tyrosine kinase signalling and widely implicated in actin cytoskeleton reorganization. Most notably, ablation of chimaerin and Nck genes in mice leads to similar phenotypes [2] , [21] . Nck adaptors have three SH3 domains in tandem (SH3-1, SH3-2 and SH3-3) and a single C-terminal SH2 domain [22] , [23] , [24] . The Nck1-binding site in α2-chimaerin is located within the first 183 amino acids, and α1-chimaerin, which lacks the SH2 domain, fails to interact with Nck1 (ref. 2 ). The specific motifs in chimaerins involved in the association with Nck1 still need to be determined. In the present study, we identify an atypical Pro-rich motif in chimaerins involved in Nck1 binding. Unlike most interactions that involve the first or second SH3 domain in Nck1, the Pro-rich motif in chimaerins interacts with the third Nck1 SH3 domain. This association occurs in response to stimulation of growth factor receptors such as EGFR and mediates β2-chimaerin activation. α2- and β2-chimaerins interact with Nck1 Recent studies found that the adaptor protein Nck1 interacts with α2-chimaerin [2] , [21] . In order to map the domains in α2-chimaerin implicated in this association, we first generated α2-chimaerin truncated mutants ( Fig. 1a ) and examined their ability to bind Nck1 using pull-down assays. Nck1 associated with wt α2-chimaerin, as well as with a GAP-deleted mutant (Δ255-433-α2-chimaerin). On the other hand, deletion of the first 128 amino acids that comprise the SH2 domain (Δ1–128-α2-chimaerin) abolished the association with Nck1. Unexpectedly, a mutant lacking the first 44 amino acids (Δ1–44-α2-chimaerin), which retains the SH2 domain, failed to interact with Nck1 ( Fig. 1b , left panel). No interaction of α2-chimaerin with glutathione S- transferase (GST) alone could be detected (data not shown). These results were confirmed by co-immunoprecipitation (co-IP) of endogenous Nck1. ( Fig. 1b , right panel). Therefore, the interaction with Nck1 is not mediated by the α2-chimaerin SH2 domain but rather involves a region upstream of the SH2 domain. 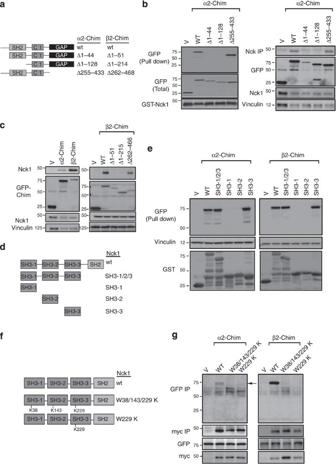Figure 1: Interaction of the α2- and β2-chimaerin N-terminal domain with the Nck1 SH3-3 domain. (a) Schematic representation of α2- and β2-chimaerin mutants. (b)Left panel, extracts from COS-1 expressing GFP-α2-chimaerin (wt or mutants) were incubated with GST-Nck1 and pulled down with glutathione Sepharose 4B beads. Levels of chimaerins in the GST precipitates were determined with an anti-GFP antibody.Right panel, extracts of COS-1 cells expressing α2-chimaerin (wt or mutant) were subject to IP with an anti-GFP antibody. Endogenous Nck1 was detected in the IP by western blot. (c)Left panel, preferential association of β2-chimaerin with endogenous Nck1.Right panel, extracts of COS-1 cells expressing β2-chimaerin (wt or mutant) were subject to IP with an anti-GFP antibody. Endogenous Nck1 was detected in the IP by western blot. (d) Schematic representation of Nck1-deleted mutants. (e) COS-1 cells expressing GFP-α2-chimaerin (left panel) or GFP-β2-chimaerin (right panel) were incubated with GST, GST-Nck1 or the indicated GST-Nck1 mutants. After pull-down, levels of chimaerins in the GST precipitates were determined with an anti-GFP antibody. (f) Schematic representation of Nck1 SH3 domain point mutants. (g) COS-1 cells were co-transfected with pEGFP-α2-chimaerin (left panel) or pEGFP-β2-chimaerin (right panel), together with plasmids encoding myc-tagged Nck1 (wt or mutants). Twenty-four hours later, cells were subject to IP with an anti-myc tag antibody. α2- and β2-chimaerins in the IP (arrow) were detected by western blot using an anti-GFP antibody. In all panels, similar results were observed in at least three independent experiments. Figure 1: Interaction of the α2- and β2-chimaerin N-terminal domain with the Nck1 SH3-3 domain. ( a ) Schematic representation of α2- and β2-chimaerin mutants. ( b ) Left panel , extracts from COS-1 expressing GFP-α2-chimaerin (wt or mutants) were incubated with GST-Nck1 and pulled down with glutathione Sepharose 4B beads. Levels of chimaerins in the GST precipitates were determined with an anti-GFP antibody. Right panel , extracts of COS-1 cells expressing α2-chimaerin (wt or mutant) were subject to IP with an anti-GFP antibody. Endogenous Nck1 was detected in the IP by western blot. ( c ) Left panel , preferential association of β2-chimaerin with endogenous Nck1. Right panel , extracts of COS-1 cells expressing β2-chimaerin (wt or mutant) were subject to IP with an anti-GFP antibody. Endogenous Nck1 was detected in the IP by western blot. ( d ) Schematic representation of Nck1-deleted mutants. ( e ) COS-1 cells expressing GFP-α2-chimaerin ( left panel ) or GFP-β2-chimaerin ( right panel ) were incubated with GST, GST-Nck1 or the indicated GST-Nck1 mutants. After pull-down, levels of chimaerins in the GST precipitates were determined with an anti-GFP antibody. ( f ) Schematic representation of Nck1 SH3 domain point mutants. ( g ) COS-1 cells were co-transfected with pEGFP-α2-chimaerin ( left panel ) or pEGFP-β2-chimaerin ( right panel ), together with plasmids encoding myc-tagged Nck1 (wt or mutants). Twenty-four hours later, cells were subject to IP with an anti-myc tag antibody. α2- and β2-chimaerins in the IP ( arrow ) were detected by western blot using an anti-GFP antibody. In all panels, similar results were observed in at least three independent experiments. Full size image Given the high homology between α2- and β2-chimaerins, we next examined if Nck1 also interacts with β2-chimaerin. Co-IP experiments shown in Fig. 1c (left panel) revealed that the amount of endogenous Nck1 recovered in β2-chimaerin IPs is much larger than in α2-chimaerin IPs, suggesting a preferential association with β2-chimaerin. Deletion mutants equivalent as those in α2-chimaerin were then generated for β2-chimaerin and tested for their ability to co-IP with endogenous Nck1. Complete loss of Nck1 binding could be observed with mutants Δ1-214-β2-chimaerin (SH2 domain deleted) or with Δ1-51-β2-chimaerin (SH2 domain intact). On the other hand, deletion of the C-terminal GAP domain (Δ262-466-β2-chimaerin) did not affect binding to Nck1 ( Fig. 1c , right panel). Taken together, these results determined that the SH2 domain in chimaerins is dispensable for the interaction with Nck1 and map the region responsible for this association near the N-terminal end. Chimaerins bind to the third SH3 domain in Nck1 The adaptor protein Nck1 contains three SH3 domains in tandem capable of binding Pro-rich regions, and a single SH2 domain implicated in phosphotyrosine binding [22] , [24] . As chimaerins do not get tyrosine phosphorylated in response to receptor activation [25] (A.G-U. and M.G.K., unpublished data) we speculated that SH3 domains in Nck1 might be involved in the association. COS-1 cell lysates expressing either α2- or β2-chimaerin were incubated with GST-Nck1 (wt), GST fused to each individual SH3 domain (SH3-1, SH3-2 or SH3-3), or GST fused to the three SH3 domains in tandem (SH3-1/2/3) ( Fig. 1d ). Interestingly, whereas SH3-1 or SH3-2 domains failed to bind chimaerins, GST-SH3-3 domain or GST-SH3-1/2/3 efficiently pulled down chimaerins ( Fig. 1e ). This was unexpected as most known Nck1-interacting proteins preferentially bind to SH3-1 or SH3-2 domains. To further establish the involvement of the Nck1 SH3-3 domain in the interaction with chimaerins, we used a co-IP assay. COS-1 cells were co-transfected with plasmids coding for α2- or -β2-chimaerin, together with myc-tagged wt Nck1 or Nck1 SH3 domain mutants where a conserved Trp was replaced by Lys ( Fig. 1f ). Trp→Lys mutations in Nck1 SH3 domains are known to abolish their interaction with Pro-rich partners [26] . Again, these co-IP assays also revealed a stronger association with β2-chimaerin than with α2-chimaerin ( Fig. 1g ). A triple SH3 domain mutant (W38K in SH3-1, W143K in SH3-2 and W229K in SH3-3) failed to associate with chimaerins. Moreover, a single mutant in the SH3-3 domain (W229K) was sufficient to abrogate the interaction. The specific involvement of the third Nck1 SH3 domain was strongly suggestive of an atypical interaction with chimaerins. An atypical Pro-rich domain mediates association with Nck1 SH3 domains are protein–protein interaction modules that recognize Pro-rich regions, typically the motif PxxP. Although sequence analysis of amino acids 1–44 and 1–54 in α2- and β2-chimaerin, respectively, did not reveal any characteristic PxxP consensus, there are two clusters containing two Pro residues each ( Fig. 2a ). To establish if any of these clusters could be implicated in Nck1 binding, we generated a series of Pro→Ala mutants both in α2- and β2-chimaerins. A GST pull-down assay revealed that double Pro mutations in the first Pro cluster (Pro 13 /Pro 14 and Pro 23 /Pro 24 in α2- and β2-chimaerin, respectively) did not affect the interaction with Nck1 ( Fig. 2b ). On the other hand, a major loss in the association with Nck1 occurred when Pro 28 /Pro 30 in α2-chimaerin or Pro 38 /Pro 40 in β2-chimaerin were mutated to Ala. We also generated triple Ala mutants for the second Pro cluster and a Pro located near this cluster. The interaction was abolished in the triple Ala mutants for Pro 28 /Pro 30 /Pro 43 in α2-chimaerin or Pro 38 /Pro 40 /Pro 53 in β2-chimaerin. These results were also confirmed by co-IP of endogenous Nck1 (see Fig. 3b below). 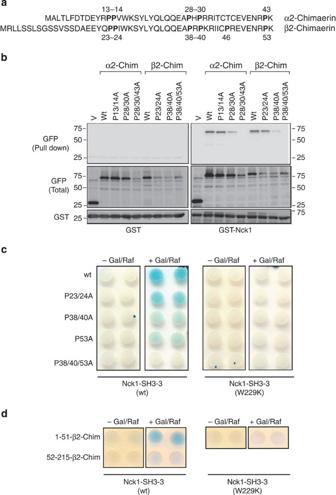Figure 2: Identification of an atypical Pro-rich region in α2- and β2-chimaerin. (a) Alignment of α2- and β2-chimaerin N-terminal regions. (b) Extracts from COS-1 cells expressing GFP-α2- or GFP-β2-chimaerin (wt or Pro→Ala mutants) were incubated with GST (left panel) or GST-Nck1 (right panel). Chimaerins in GST precipitates were detected by western blot with an anti-GFP antibody. (c) Association by yeast two-hybrid between wild-type or mutated β2-chimaerin (amino acids 1–186) and SH3-3-Nck1 Wt or W229K mutant.Gal/Raf, galactosidase/raffinose. (d) Interaction between the N-terminal region of β2-chimaerin (amino acids 1–53) and SH3-3-Nck1. In all panels, similar results were observed in at least three independent experiments. Figure 2: Identification of an atypical Pro-rich region in α2- and β2-chimaerin. ( a ) Alignment of α2- and β2-chimaerin N-terminal regions. ( b ) Extracts from COS-1 cells expressing GFP-α2- or GFP-β2-chimaerin (wt or Pro→Ala mutants) were incubated with GST ( left panel ) or GST-Nck1 ( right panel ). Chimaerins in GST precipitates were detected by western blot with an anti-GFP antibody. ( c ) Association by yeast two-hybrid between wild-type or mutated β2-chimaerin (amino acids 1–186) and SH3-3-Nck1 Wt or W229K mutant. Gal/Raf , galactosidase/raffinose. ( d ) Interaction between the N-terminal region of β2-chimaerin (amino acids 1–53) and SH3-3-Nck1. In all panels, similar results were observed in at least three independent experiments. 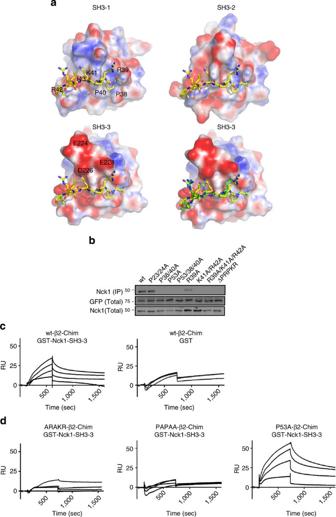Figure 3: Basic amino acids in the Pro-rich region of β2-chimaerin mediate the interaction with Nck1 SH3-3. (a) Analysis of binding interfaces between the third Nck1 domain (SH3-3) and the Pro-rich motif PRPKR (β2-chimaerin).White=neutral charge;red=negative charge;blue=positive charge;yellow=PRPKR (β2-chimaerin);green=PHPRR (α2-chimaerin). (b) COS-1 cells were transfected with pEGFP plasmids encoding wt-β2-chimaerin or various mutated forms of β2-chimaerin. After 24 h, cell extracts were subject to IP with an anti-GFP antibody. Nck1 in the IP were detected by western blot. Two additional experiments gave similar results. (c) Representative Biacore sensorgrams showing the interaction between immobilized GST-Nck1 SH3-3 or GST alone and increasing concentrations (1, 10, 20, 40 μM) of wild-type β2-chimaerin N-terminal peptides. (d) Representative Biacore sensorgrams showing the interaction between immobilized GST-Nck1 SH3-3 and increasing concentrations (1, 10, 20, 40 μM) of mutated β2-chimaerin N-terminal peptides. Full size image Figure 3: Basic amino acids in the Pro-rich region of β2-chimaerin mediate the interaction with Nck1 SH3-3. ( a ) Analysis of binding interfaces between the third Nck1 domain (SH3-3) and the Pro-rich motif PRPKR (β2-chimaerin). White =neutral charge; red =negative charge; blue =positive charge; yellow =PRPKR (β2-chimaerin); green =PHPRR (α2-chimaerin). ( b ) COS-1 cells were transfected with pEGFP plasmids encoding wt-β2-chimaerin or various mutated forms of β2-chimaerin. After 24 h, cell extracts were subject to IP with an anti-GFP antibody. Nck1 in the IP were detected by western blot. Two additional experiments gave similar results. ( c ) Representative Biacore sensorgrams showing the interaction between immobilized GST-Nck1 SH3-3 or GST alone and increasing concentrations (1, 10, 20, 40 μM) of wild-type β2-chimaerin N-terminal peptides. ( d ) Representative Biacore sensorgrams showing the interaction between immobilized GST-Nck1 SH3-3 and increasing concentrations (1, 10, 20, 40 μM) of mutated β2-chimaerin N-terminal peptides. Full size image To validate the requirement of the second Pro cluster in the association with Nck1, we used a yeast two-hybrid approach. pLexA vectors encoding the N-terminal domain of β2-chimaerin (amino acids 1–186) or corresponding mutants P23/24A, P38/40A, P53A or P38/40/53A were cotransformed, together with pB42AD vectors encoding either wt SH3-3-Nck1 or W229K-SH3-3-Nck1 (HA tagged) into EGY48 yeast containing p8OP-LacZ vector [27] . A strong interaction was observed between β2-chimaerin and wt Nck1 SH3-3. Mutation of Trp 229 in the Nck1 SH3-3 domain abolished the interaction. Moreover, the interaction was impaired by mutation of Pro 38 /Pro 40 but essentially unaffected by mutation of Pro 23 /Pro 24 ( Fig. 2c ). These results authenticate the involvement of the second Pro cluster in the association with Nck1 and also indicate that the interaction is direct. To further rule out the involvement of the SH2 domain in β2-chimaerin, we generated two additional pLexA constructs, one comprising the first 53 amino acids and lacking the SH2 domain (1-51-β2-chimaerin) and the other comprising only the SH2 domain (52-215-β2-chimaerin). The yeast two-hybrid assay revealed a strong interaction with 1-51-β2-chimaerin but no interaction at all with 52-215-β2-chimaerin. As expected, the mutated SH3-3 domain (W229K) failed to interact with 1-51-β2-chimaerin ( Fig. 2d ). Essential role of basic residues in interaction with Nck1 To gain structural insight into the Nck1 interaction with chimaerins, we generated models of Nck1 SH3-3 in complex with the second Pro cluster of α2- and β2-chimaerins. The solution structure (NMR) of the SH3-3 domain of human Nck2 was used to build a homology model of the Nck1 SH3-3 domain. The Pro-rich region in chimaerins is rich in basic amino acids (see Fig. 2a ). A close analysis of the β2-chimaerin-SH3-3 interface shows that the side chains of Arg 39 , Lys 41 and Arg 42 in the PRPKR motif are oriented towards the binding cleft of the SH3 domain ( Fig. 3a ). In α2-chimaerin, His 29 replaces Arg 39 , Arg 31 replaces Lys 41 (PHPRR motif) and Arg 32 is not facing the binding cleft. Comparison of electrostatic potential surfaces provided interesting insights into the differential involvement of Nck1 SH3 domains. Nck1 SH3-3 has a negatively charged surface made up of residues Asp 226 and Glu 228 that complement basic-charged residues Arg 39 , Lys 41 and Arg 42 . On the other hand, the surface of SH3-1 is mostly positively charged, and SH3-2 has almost equal positive and negative charge distribution. Thus, electrostatic potential seems critical in driving the interaction between Nck1 SH3-3 and chimaerins. To validate this model experimentally, we generated Arg/Lys→Ala mutants in β2-chimaerin: single mutant R39A, double mutant K41A/R42A and triple mutant R39A/K41A/R42A. Notably, a substantial reduction in the association with endogenous Nck1 was observed in the co-IP assays, particularly with the double and triple mutants ( Fig. 3b ). In agreement with pull-downs and yeast two-hybrid assays, co-IP assays also show that mutation of Pro 38 /Pro 40 to Ala in β2-chimaerin abolished the interaction with Nck1, whereas Pro 23 /Pro 24 were dispensable. A five amino acid deletion mutant (ΔPRPKR-β2-chimaerin) also failed to co-IP with Nck1. Altogether, our results determined the minimum Nck1-binding motif in β2-chimaerin as PRPKR. We noted in this analysis that mutation of Pro 53 in β2-chimaerin, which is close to the primary Nck1-binding motif, also prevented the association with Nck1. Next, we examined binding interactions of β2-chimaerin to immobilized GST-Nck1 SH3-3 domain using surface plasmon resonance (SPR). A peptide comprising amino acids 34–59, that includes the second Pro-rich cluster, was generated. After flowing different concentrations of the peptide, data collected from sensorgrams revealed a dissociation constant ( K D ) of 18±10 μM (n=6). The wild-type peptide did not bind to immobilized GST alone ( Fig. 3c ). A longer version of the peptide gave a similar K D (8±6 μM, n =6, Supplementary Fig. S1 ). When we run similar experiments with a peptide with basic amino acids in the PRPKR domain mutated to Ala (PAPAA-β2-chim), binding could not be detected. Similarly, mutation of Pro residues in this domain (ARAKR-β2-chim) markedly reduced binding. Unlike the pull-down experiments, mutation of Pro 53 to Ala in the peptide (P53A-β2-chim) did not affect binding ( K D =3±2 μM, n =3) ( Fig. 3d ). Thus, Pro 53 may not be directly involved in the association with the SH3-3 domain, as predicted from the modelling ( Supplementary Fig. S2 ). As Pro 53 is located just before the start of the SH2 domain, one possibility is that introducing an Ala in that position may alter the protein conformation and indirectly affect binding to Nck1. Nck1 interacts with membrane-bound β2-chimaerin The SH3-3 domain of Nck1 was docked onto the Pro-rich region in the conformation observed in the structure of full-length β2-chimaerin that we previously solved [20] . In the docked model, the Nck1 SH3-3 domain is lodged in a broad fork between the SH2 and Rac-GAP domains of β2-chimaerin, and has steric clashes with the αN helix and the SH2 domain ( Figs 4a ). Therefore, interaction of Nck1 SH3-3 with the PRPKR motif is not possible without significant structural rearrangements in the closed conformation of chimaerins. Structural rearrangements of the same region had been predicted for DAG binding to the pocket on the surface of the C1 domain and subsequent activation of β2-chimaerin [20] . We, therefore, concluded that the SH3-3 domain in Nck1 can only bind to the open, active conformation of β2-chimaerin. As predicted from this analysis, a physical interaction could not be observed between purified β2-chimaerin and the SH3-3 domain of Nck1 by size-exclusion chromatography ( Supplementary Fig. S3 ). 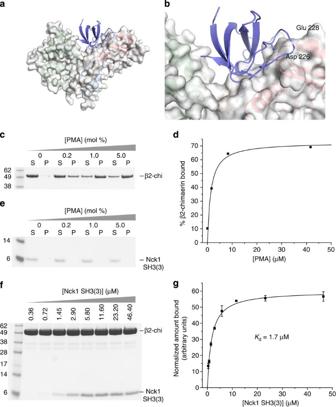Figure 4: The interaction between β2-chimaerin and Nck1 depends on the membrane-bound conformation of β2-chimaerin. (a) Docking model of β2-chimaerin and Nck1 SH3-3 to show that steric clash makes binding of Nck-SH3 to the closed state of β2-chimaerin unfavourable. β2-chimaerin is shown as ribbon and translucent surface. Nck1 SH3-3 is shown as purple ribbon. (b) Enhanced view ofa. (c) β2-chimaerin binding to PMA-containing SLVs.S=supernatant fraction,P=pellet fraction. (d) Binding curve for PMA-dependent recruitment of β2-chimaerin. (e) Nck1 SH3-3 binding to PMA-containing SLVs. (f) Corecruitment of Nck1 SH3-3 and β2-chimaerin to PMA-containing SLVs. (g) Binding curve for Nck1 SH3-3 interaction with β2-chimaerin gives aKD=1.7 μM. Results are the mean±s.d. of three experiments. Figure 4: The interaction between β2-chimaerin and Nck1 depends on the membrane-bound conformation of β2-chimaerin. ( a ) Docking model of β2-chimaerin and Nck1 SH3-3 to show that steric clash makes binding of Nck-SH3 to the closed state of β2-chimaerin unfavourable. β2-chimaerin is shown as ribbon and translucent surface. Nck1 SH3-3 is shown as purple ribbon. ( b ) Enhanced view of a . ( c ) β2-chimaerin binding to PMA-containing SLVs. S =supernatant fraction, P =pellet fraction. ( d ) Binding curve for PMA-dependent recruitment of β2-chimaerin. ( e ) Nck1 SH3-3 binding to PMA-containing SLVs. ( f ) Corecruitment of Nck1 SH3-3 and β2-chimaerin to PMA-containing SLVs. ( g ) Binding curve for Nck1 SH3-3 interaction with β2-chimaerin gives a K D =1.7 μM. Results are the mean±s.d. of three experiments. Full size image To investigate whether the interaction between β2-chimaerin and Nck1 depends on the membrane-bound conformation of β2-chimaerin, we used an in vitro sucrose-loaded vesicles (SLV) pelleting assay in the presence of the DAG mimetic phorbol 12-myristate 13-acetate (PMA). β2-chimaerin binds to SLVs in a PMA-dependent manner ( Figs 4c ). We could not detect binding of Nck1 SH3-3 to the same vesicles either in the absence or presence of PMA ( Fig. 4e ). Interestingly, Nck1 SH3-3 could be recruited to SLVs in a PMA- and β2-chimaerin-dependent manner. To determine the binding of Nck1 SH3-3 to β2-chimaerin-bound SLVs more accurately, SLVs containing 5 mol% PMA were incubated with different concentrations of Nck1 SH3-3 in the presence of β2-chimaerin. As shown in Figs 4f , Nck1 SH3-3 binds to PMA-containing SLVs in a β2-chimaerin-dependent manner, with a K D =1.7 μM. DAG-dependent association of β2-chimaerin with Nck1 We have previously shown that α2- and β2-chimaerins translocate to the plasma membrane in response to EGF, where they associate with active Rac1 to promote GTP hydrolysis from this small G-protein. This relocalization is mediated by DAG, a product of PIP 2 hydrolysis by PLCγ that is transiently generated upon EGFR receptor stimulation. Deletion of the C1 domain (the DAG-binding domain) or mutations that disrupt its conformation abrogate the translocation of α2- and β2-chimaerins and their association with Rac1 in response to growth factors [5] , [9] , [17] . Nck1 also recruits to growth factor receptors (including EGFR) upon their stimulation [28] . We hypothesized that EGF induces the association of β2-chimaerin and Nck1 at the plasma membrane. Co-IP assays revealed that EGF promotes the formation of a complex between endogenous Nck1 and β2-chimaerin in COS-1 cells ( Fig. 5a ). To further confirm this interaction in cells we developed a fluorescence resonance energy transfer (FRET) assay ( Fig. 5b , see also Supplementary Fig. S4 ) employing an approach similar to that previously used for the analysis of the dynamic interaction of β2-chimaerin and Rac1 (ref. 9 ). CFP-Nck1 and YFP-β2-chimaerin were expressed in COS-7 cells, and time-dependent changes in FRET were determined in response to EGF treatment. EGF caused a significant FRET response in the cell periphery. The EGFR inhibitor AG1478 abolished this effect ( Fig. 5c ). Changes in FRET in the cytosolic compartment were negligible, suggesting that intracellular relocalization of β2-chimaerin to the plasma membrane is required in order to interact with Nck1 ( Fig. 5d ). We were unable to detect changes in FRET in response to EGF in cells expressing the pairs CFP-Nck1/YFP, CFP/YFP-β2-chimaerin or CFP/YFP (see Supplementary Fig. S5 ). 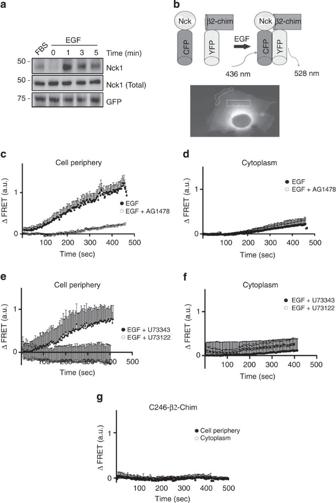Figure 5: EGF promotes the interaction between β2-chimaerin and Nck1 in a DAG-dependent manner. (a) COS-1 cells expressing GFP-β2-chimaerin were serum-starved for 24 h and treated with EGF (100 ng ml−1). Cell extracts were subject to IP with an anti-GFP antibody. Nck1 was detected in the IP using an anti-Nck antibody.Lane 1, cells growing in medium with 10% fetal bovine serum. (b) Schematic representation of the FRET assay to assess Nck1-β2-chimaerin interaction in cells. Typical peripheral and cytoplasmatic cell sections selected for analysis are shown. (c) FRET in peripheral cellular sections was measured every 3 s after EGF treatment (100 ng ml−1), both in the absence and presence of the EGFR inhibitor AG1478 (1 μM). (d) FRET in cytoplasmatic cellular sections after EGF treatment, both in the absence and presence of AG1478. (e) and (f) FRET in cell peripheral (e) and cytoplasmatic (f) sections after EGF treatment in the presence of either U73122 or its inactive analogue U73343 (10 μM, added 30 min before and during EGF treatment). (g) FRET in peripheral and cytoplasmatic sections using the pair CFP-Nck1 and YFP-C246A-β2-chimaerin. For all FRET experiments, data are expressed as mean±s.e.m. of 6–13 cells. a.u., arbitrary unit. Figure 5: EGF promotes the interaction between β2-chimaerin and Nck1 in a DAG-dependent manner. ( a ) COS-1 cells expressing GFP-β2-chimaerin were serum-starved for 24 h and treated with EGF (100 ng ml −1 ). Cell extracts were subject to IP with an anti-GFP antibody. Nck1 was detected in the IP using an anti-Nck antibody. Lane 1 , cells growing in medium with 10% fetal bovine serum. ( b ) Schematic representation of the FRET assay to assess Nck1-β2-chimaerin interaction in cells. Typical peripheral and cytoplasmatic cell sections selected for analysis are shown. ( c ) FRET in peripheral cellular sections was measured every 3 s after EGF treatment (100 ng ml −1 ), both in the absence and presence of the EGFR inhibitor AG1478 (1 μM). ( d ) FRET in cytoplasmatic cellular sections after EGF treatment, both in the absence and presence of AG1478. ( e ) and ( f ) FRET in cell peripheral ( e ) and cytoplasmatic ( f ) sections after EGF treatment in the presence of either U73122 or its inactive analogue U73343 (10 μM, added 30 min before and during EGF treatment). ( g ) FRET in peripheral and cytoplasmatic sections using the pair CFP-Nck1 and YFP-C246A-β2-chimaerin. For all FRET experiments, data are expressed as mean±s.e.m. of 6–13 cells. a.u., arbitrary unit. Full size image As DAG mediates EGF-induced translocation of β2-chimaerin and its association with Rac1 (ref. 9 ), we next examined if DAG is also necessary for the β2-chimaerin–Nck1 interaction. We found that EGF-induced FRET in the cell periphery was substantially lower when cells were pretreated with the PLC inhibitor U73122 as compared with its inactive analogue U73343 ( Figs 5e ). Also, the DAG-unresponsive C1 domain mutant C246A-β2-chimaerin failed to translocate to the membrane or to interact with Rac1 upon EGFR stimulation [9] , [15] . Unlike wt YFP-β2-chimaerin, YFP-C246A-β2-chimaerin was unable to generate peripheral FRET in response to EGF when coexpressed with CFP-Nck1 ( Fig. 5g ). Thus, translocation of β2-chimaerin to the cell periphery is mediated by DAG binding to the C1 domain is required for the association with Nck1. Translocation of β2-chimaerin by EGF requires Nck1 One attractive possibility is that Nck1 is required for the activation of chimaerins by EGFR. We generated β2-chimaerin mutants in Pro-rich domains and examined their ability to associate with Nck1 in response to EGF using FRET. Whereas a mutant of the first Pro-rich cluster (YFP-P23/24A-β2-chimaerin) behaved essentially as wild-type YFP-β2-chimaerin, mutation in the second Pro-rich cluster (YFP-P38/40A-β2-chimaerin) failed to give a FRET response ( Fig. 6a and Supplementary Fig. S4 ), as also observed with the mutant YFP-P53A-β2-chimaerin ( Supplementary Fig. S6 ). We also took advantage of W308K-Nck1, an SH2 domain mutant unable to bind EGFR upon receptor stimulation [24] . Using the FRET approach described above we found that CFP-W308K-Nck1 was unable to associate with YFP-β2-chimaerin in the cell periphery in response to EGF. As expected, the SH3-3 domain mutant W229K also failed to give a FRET response upon EGFR stimulation ( Fig. 6b ). As a third strategy we used a FRET approach with pairs CFP-Rac1 and YFP-β2-chimaerin ( Fig. 6c ), as previously described [9] , using Nck-depleted cells. A dual Nck1/Nck2 knockdown approach was considered in order to avoid any potential compensatory effects by the highly homologous Nck2. Validated RNAi duplexes designed to silence human Nck1/Nck2 caused a nearly complete depletion in monkey-derived COS-7 cells ( Fig. 6d ) due to high sequence homology (unpublished data). As we previously reported [9] , EGF caused a time-dependent peripheral FRET signal between CFP-Rac1 and YFP-β2-chimaerin ( Fig. 6e ). Notably, this effect was significantly reduced in Nck-depleted cells ( Fig. 6f ). Thus, Nck is required for the ability of β2-chimaerin to bind its target Rac1 at the plasma membrane. 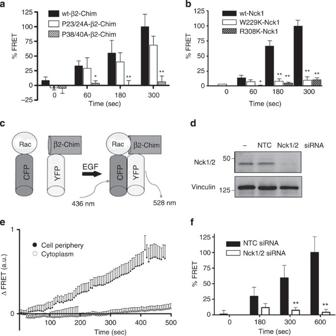Figure 6: Nck is required for β2-chimaerin activation by EGF. (a) FRET between YFP-β2-chimaerin (wt, and mutants P23/24A and P38/40A) and CFP-Nck1 after treatment of COS-7 cells with EGF (100 ng ml−1). Data (mean±s.e.m.) are expressed as % of maximum FRET with wt YFP-β2-chimaerin (analysis of variance test with Bonferroni adjustment was used; *P<0.05; **P<0.01;n=10). (b) FRET between YFP-β2-chimaerin and CFP-Nck1 (wt, W229K or W308K) after treatment of COS-7 cells with EGF (100 ng ml−1). Data (mean±s.e.m.) are expressed as % of maximum FRET with wt CFP-Nck1 (analysis of variance test with Bonferroni adjustment was used; *P<0.05; **P<0.01;n=10). (c) Schematic representation of the FRET assay to assess Rac1-β2-chimaerin association (adapted from ). (d) Depletion of Nck1/2 in COS-7 cells using RNAi, as determined 48 h after transfection.NTC, non-target control siRNA. (e) FRET analysis in COS-7 cells expressing CFP-Rac1 and YFP-β2-chimaerin was measured every 6 s after EGF treatment, both in peripheral and cytoplasmatic sections. Data are expressed as mean±s.e.m. (n=10). (f) FRET in response to EGF in the periphery of cells transfected with eitherNTCor Nck1/2 RNAi. Data (mean±s.e.m.) are expressed as percentage of maximum FRET with wt YFP-β2-chimaerin (unpaired Student’st-test was used; *P<0.05; **P<0.01;n=10). a.u., arbitrary unit. Figure 6: Nck is required for β2-chimaerin activation by EGF. ( a ) FRET between YFP-β2-chimaerin (wt, and mutants P23/24A and P38/40A) and CFP-Nck1 after treatment of COS-7 cells with EGF (100 ng ml −1 ). Data (mean±s.e.m.) are expressed as % of maximum FRET with wt YFP-β2-chimaerin (analysis of variance test with Bonferroni adjustment was used; * P <0.05; ** P <0.01; n =10). ( b ) FRET between YFP-β2-chimaerin and CFP-Nck1 (wt, W229K or W308K) after treatment of COS-7 cells with EGF (100 ng ml −1 ). Data (mean±s.e.m.) are expressed as % of maximum FRET with wt CFP-Nck1 (analysis of variance test with Bonferroni adjustment was used; * P <0.05; ** P <0.01; n =10). ( c ) Schematic representation of the FRET assay to assess Rac1-β2-chimaerin association (adapted from ). ( d ) Depletion of Nck1/2 in COS-7 cells using RNAi, as determined 48 h after transfection. NTC , non-target control siRNA. ( e ) FRET analysis in COS-7 cells expressing CFP-Rac1 and YFP-β2-chimaerin was measured every 6 s after EGF treatment, both in peripheral and cytoplasmatic sections. Data are expressed as mean±s.e.m. ( n =10). ( f ) FRET in response to EGF in the periphery of cells transfected with either NTC or Nck1/2 RNAi. Data (mean±s.e.m.) are expressed as percentage of maximum FRET with wt YFP-β2-chimaerin (unpaired Student’s t -test was used; * P <0.05; ** P <0.01; n =10). a.u., arbitrary unit. Full size image Evidence for a dual input for β2-chimaerin activation Although DAG is essential for EGF-induced activation of α2- and β2-chimaerins, by itself this lipid only poorly activates chimaerins unless supraphysiological concentrations are used. Likewise, phorbol esters fail to translocate chimaerins up to micromolar concentrations [15] . A conformational rearrangement in chimaerins is required to expose the C1 domain [5] , [17] , [20] . We speculated that a signal independent of PLCγ-DAG contributes to the translocation and activation of chimaerins via Nck1. We had previously noticed that the tyrosine phosphatase inhibitor sodium pervanadate caused a marked potentiation of PMA-induced translocation of α2-chimaerin from a soluble to a particulate fraction (EC 50 −pervanadate ~1 μM; EC 50 +pervanadate=10 nM) (see Supplementary Fig. S7a ). SH2 domain mutants with impaired phosphotyrosine binding [19] , [29] were sensitized to PMA-induced translocation by sodium pervanadate treatment in a manner similar to wt α2-chimaerin (see Supplementary Fig. S7b ), arguing that the SH2 domain does not mediate translocation. When we examined the intracellular redistribution of GFP-β2-chimaerin by fluorescence microscopy we noticed that PMA (10 nM) failed to cause an obvious translocation; however, GFP-β2-chimaerin could be readily observed at the cell periphery in response to PMA after pretreatment with sodium pervanadate ( Fig. 7a , see also Supplementary Fig. S8 ). Notably, when we carried out similar experiments in Nck-depleted cells, we were unable to observe any obvious redistribution of GFP-β2-chimaerin by PMA/pervanadate ( Figs 7a ). Therefore, a tyrosine phosphorylation-dependent mechanism facilitates the activation of chimaerins, and this redistribution requires Nck. 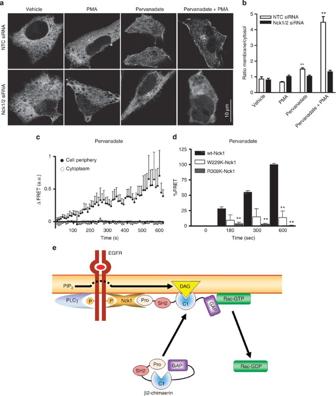Figure 7: Nck is required for β2-chimaerin activation by sodium pervanadate. (a) COS-7 cells were transfected with pEGFP-β2-chimaerin and either Nck1/2 or non-target control (NTC) siRNA. After 48 h, cells were treated with PMA (10 nM, 15 min) either in the absence or presence of sodium pervanadate (1 mM, 15 min before and during PMA), and visualized by confocal microscopy. Representative micrographs are shown. (b) Quantification of translocation using ImageJ. Data are expressed as mean±s.e.m. of 7–15 individual cells for each group. (unpaired Student’st-test was used; **P<0.01 versus NTC siRNA).NTC, non-target control. (c) FRET analysis in COS-7 cells expressing CFP-Nck1 and YFP-β2-chimaerin was measured after sodium pervanadate treatment, both in peripheral and cytoplasmatic sections. Data are expressed as mean±s.e.m. (n=10). (d) FRET between YFP-β2-chimaerin and Nck1 (wt, W229K or W308K) at different times after treatment with sodium pervanadate (1 mM). Data (mean±s.e.m.) are expressed as percentage of maximum FRET with wt YFP-β2-chimaerin (analysis of variance test with Bonferroni adjustment was used; *P<0.05; **P<0.01;n=10). (e) Model for EGFR-mediated regulation of β2-chimaerin via DAG and Nck1. Scale bar, 10 μm. a.u., arbitrary unit. Figure 7: Nck is required for β2-chimaerin activation by sodium pervanadate. ( a ) COS-7 cells were transfected with pEGFP-β2-chimaerin and either Nck1/2 or non-target control ( NTC ) siRNA. After 48 h, cells were treated with PMA (10 nM, 15 min) either in the absence or presence of sodium pervanadate (1 mM, 15 min before and during PMA), and visualized by confocal microscopy. Representative micrographs are shown. ( b ) Quantification of translocation using ImageJ. Data are expressed as mean±s.e.m. of 7–15 individual cells for each group. (unpaired Student’s t -test was used; ** P <0.01 versus NTC siRNA). NTC , non-target control. ( c ) FRET analysis in COS-7 cells expressing CFP-Nck1 and YFP-β2-chimaerin was measured after sodium pervanadate treatment, both in peripheral and cytoplasmatic sections. Data are expressed as mean±s.e.m. ( n =10). ( d ) FRET between YFP-β2-chimaerin and Nck1 (wt, W229K or W308K) at different times after treatment with sodium pervanadate (1 mM). Data (mean±s.e.m.) are expressed as percentage of maximum FRET with wt YFP-β2-chimaerin (analysis of variance test with Bonferroni adjustment was used; * P <0.05; ** P <0.01; n =10). ( e ) Model for EGFR-mediated regulation of β2-chimaerin via DAG and Nck1. Scale bar, 10 μm. a.u., arbitrary unit. Full size image Finally, we examined the effect of sodium pervanadate on FRET in cells coexpressing pairs YFP-β2-chimaerin and CFP-Nck1. Treatment with sodium pervanadate caused a significant activation of EGFR [30] . Notably, sodium pervanadate produced a FRET response using the pairs YFP-β2-chimaerin and CFP-Nck1 ( Fig. 7c ). This response could not be detected when CFP-W308K-Nck1 or CFP-W229K-Nck1 were used ( Fig. 7d ), as shown with EGF (see Fig. 6b ) Taken together, these results suggest that translocation of β2-chimaerin in response to EGFR stimulation not only requires DAG but it is also dependent on Nck1. In the present study, we identified an atypical motif in the N-terminal domain of α2- and β2-chimaerins that mediates the association with Nck1, a well-established mediator of tyrosine-kinase receptors signals. An important observation in our study is that the third SH3 domain in Nck1, for which only few partners have been identified so far, mediates the association with chimaerins. More importantly, Nck1 is required for the activation of β2-chimaerin in response to EGFR stimulation. Deletion of the autoinhibitory N-terminal domain in α2- or β2-chimaerins facilitates DAG access to the C1 domain and membrane anchoring [5] , [20] , [31] . We propose that release of autoinhibition in β2-chimaerin is required to expose a docking site for Nck1 binding. While other GAPs such as p50 Rho GAP and ASAP1 are also regulated through autoinhibitory mechanisms [32] , [33] , chimaerins represent the only known example of DAG-activated GAPs regulated by a conformational switch. The SH2 domain in α2- and β2-chimaerins is not implicated in Nck1 binding, however, this domain can (at least in the case of α2-chimaerin) directly associate with EphA4 (ref. 34 ). The N-terminal region in α2- and β2-chimaerins has two clusters containing prolines, although none of them fulfills the canonical PxxP recognition motif. Only the Pro cluster displaying the motif P(R/H)P(R/K)R is capable of interacting with Nck1. Whereas most SH3 domains recognize (R/K)xxPxxP (Class I) or PxxPx (R/K) (Class II) motifs, a few have the ability to bind atypical motifs that in some cases are rich in basic amino acids or even lack Pro residues [23] , [35] , [36] , [37] . The SH3-binding motif in chimaerins does not resemble any of the known basic-rich motifs, such as the RKxxY motif in the adaptor protein SKAP-55 or the RxxK motif in the deubiquitination enzyme UBPY and Gads [38] , [39] , [40] . A feature that sets apart the chimaerin P(H/R)P(R/K)R motif from other SH3-binding motifs is its unique mode of recognition that does not involve direct contacts via Pro residues but rather engages the side chains of basic amino acids in the association with a highly acidic environment in the Nck1 SH3-3 domain. The side chains of Arg 39 , Lys 41 and Arg 42 in the β2-chimaerin/SH3-3 interface are facing the binding cleft of the SH3 domain. The reduced association of α2-chimaerin with Nck1 may be explained by the different orientation of one of the basic amino acids (Arg 32 ) that is not pointing towards the binding cleft, with only His 29 and Arg 31 (which replaces Arg 39 and Lys 41 in β2-chimaerin, respectively) facing the interface with the SH3 domain. The lack of interaction of chimaerins with SH3-1 and SH3-2 domains in Nck1 is most likely related to differences in charge distribution, as SH3-1 and SH3-2 do not display the negatively charged environment that allows for charge complementarity with basic residues in the β2-chimaerin Pro-rich motif. A structural analysis of SH3-3 domains in Nck adaptors predicted that the large negative patch could accommodate Arg and Lys residues [37] , and not surprisingly Nck1 SH3-3 has been implicated in interactions with non-canonical RxxK motifs [36] , [37] , [41] . A number of steric constrains characteristic of Nck1 SH3-3 makes this domain generally less favourable for protein–protein interactions and restricts the number of potential partners [37] . The SH3-3 domain in Nck2 has been shown to be involved in the formation of ultraweak protein–protein complexes that cannot even be detected by co-IP experiments [42] ; however, we can readily detect the association of endogenous Nck1 with β2-chimaerin in cells or biochemically. Using SPR we determined a low micromolar-binding affinity for the isolated Nck1 SH3-3 domain to a short peptide comprising the PRPKR motif, which is in the range reported for other protein interactions via SH3 domains [39] , [41] . Of note, Ger et al. [43] have recently reported that p120 Ras-GAP associates with Nck1 possibly via a Pro-rich region, and that this association may involve SH3-1 and SH3-3 domains. Thus, common regulatory mechanisms involving the Nck1 adaptor may govern the activation of GAPs for small GTPases. We propose a model of β2-chimaerin signalling that involves a dual regulation by lipid–protein and protein–protein interactions ( Fig. 7e ). DAG binding to the C1 domain is required but not sufficient for β2-chimaerin activation. The in vitro Rac-GAP activity of β2-chimaerin is slightly increased by PS vesicles at concentrations similar to those in the inner leaflet of the plasma membrane, and DAG greatly enhances β2-chimaerin binding to acidic phospholipid vesicles [17] . Thus, PS can act as a platform for β2-chimaerin activation by DAG. Based on structural analysis [20] , the activating conformational change results in the exposure of hydrophobic surfaces that bind with the plasma membrane and that are otherwise folded over the C1 domain in the close conformation. Upon stimulation by DAG, there is a shift in equilibrium towards conformers with the Pro-rich domain exposed and hence able to bind to Nck1. We postulate that this adaptor serves as a bridge between EGFR and chimaerins. Moreover, the impaired β2-chimaerin translocation and association with Rac1 by EGFR stimulation observed in Nck-depleted cells argues for a key role for Nck1 in β2-chimaerin activation. In other words, a dual input consisting of DAG generation via PLCγ and association with Nck1 may facilitate the access of β2-chimaerin to plasma membrane effectors in response to EGF. The emerging model suggests that Nck1 forms part of a multimeric complex that modulates Rac signalling. Not only chimaerin Rac-GAPs associate with Nck adaptors, but also Rac-GEFs such as Dock180 and Rac1 effectors such as Pak1 do [23] , [44] , [45] . A dynamic model may be envisioned in which guanine-nucleotide exchange factor (GEFs) and GAPs compete for Nck1 binding (for example, Dock180 and chimaerins both competing for binding to SH3-3, see Tu et al. [44] ). It is conceivable that association of β2-chimaerin with Nck adaptors is a required step for Rac inactivation, and that this event promotes the dissociation of Rac from Pak1, thus limiting Rac signalling. Our model for chimaerin activation has analogies with that recently described for PKC, despite obvious differences. Unlike chimaerins, DAG-regulated PKCs contain two C1 domains in tandem (C1a and C1b). PKCβII exists in a ‘closed’ conformation stabilized by internal contacts between the C1b domain and other regions of the protein, with which C1 domain ligands and acidic phospholipids must compete [46] . Like chimaerins, PKCβII is sensitized to PMA-induced translocation by disruption of internal contacts. PKCs also expose sites for protein–protein interaction (such as with RACKs) when they achieve the active state. Pharmacological inhibition of PKC–RACK interaction hampers PKC translocation and activation [47] , [48] . Thus, analogous lipid–protein and protein–protein interactions seem to mechanistically regulate unrelated families of C1 domain-containing proteins. It should be noted that a PxxP motif is present in DAG-regulated PKC isozymes and other AGC kinases, and it has been implicated in the association with proteins that control protein maturation and possibly in allosteric kinase activation [49] , [50] . In summary, our results established a crucial role for the β2-chimaerin PRPKR motif in binding Nck1. Stimulation of EGFR promotes a conformational rearrangement in chimaerins that releases autoinhibition and exposes this atypical Pro-rich motif in the N-terminus for binding to the SH3-3 domain in the adaptor protein. As hyperactivation of chimaerins has been linked to several diseases, we speculate that the interaction with Nck1 may have significant physiopathological implications, and that conceivably, targeting this association may have therapeutic significance. Reagents PMA was purchased from LC Laboratories (Woburn, MA). Epidermal growth factor (EGF) was obtained from Roche (Indianapolis, IN). Cell culture reagents were purchased from Invitrogen (Carlsbad, CA). U73122 and U73343 were obtained from Sigma (Saint Louis, MO). AG1478 was purchased from Calbiochem (Merck, San Diego, CA). Cell culture and transfections COS-1, COS-7 and HeLa cells (American Type Culture Collection) were cultured in Dulbecco’s modified Eagle’s medium supplemented with 10% fetal bovine serum, 100 U ml −1 penicillin, and 100 μg ml −1 streptomycin in a humidified 5% CO 2 atmosphere at 37 °C. Plasmid transfections (0.5–1.0 μg) were carried out using Lipofectamine2000 (Invitrogen, #11668-027) in 100 mm plates with cells at ~60% confluency or FuGENE6 (Roche, #11815091001). For Nck1/2 RNAi we used a SMARTpool from Dharmacon (Lafayette, CO, L-006354-00-0005/L-019547-00-0005). For RNAi transfection we used Lipofectamine RNAiMAX Transfection Reagent (Invitrogen, #13778-075). Generation of α2- and β2-chimaerin mutants Point mutants for α2- and β2- chimaerin were generated using the Quick-Change II XL s mutagenesis kit (Stratagene, La Jolla, CA), using pEGFP-C3-α2-chimaerin or pEGFP-C3-β2-chimaerin as templates. Deletion mutants were generated using standard PCR approaches, using the primers described in Supplementary Table S1 . PCR products were ligated into pCRII using the TA cloning kit (Invitrogen) and the sequence was verified by sequencing. Eco RI– Bam HI fragments were isolated from pCRII and subcloned into pEGFP-C3. Localization studies and immunofluorescence Cells were plated in glass coverslips plates and transfected with pEGFP-β2-chimaerin. After 48 h, cells were subjected to various treatments. Images were viewed using a Carl Zeiss LSM 510 laser scanning fluorescence microscope. For quantitation, we used ImageJ to estimate fluorescent intensities across one cell in a given image. The extent of membrane translocation was calculated using the ratio between average intensities in the plasma membrane and the cytoplasm. Translocation by subcellular fractionation was carried out essentially as previously described [15] , [27] . Yeast two-hybrid assays Experiments were done essentially as previously described in Wang and Kazanietz [27] . pLexA expression vectors, which contain a His marker, were cotransformed into the yeast strain EGY48, together with pB42AD-HA-tagged expression vectors, which have a Trp marker, and the p80P-LacZ reporter vector ( Ura marker). Transformants were plated on yeast dropout medium lacking Trp , Ura and His , thereby selecting for the plasmids encoding proteins capable of two-Hybrid interaction as evidenced by transactivation of the LacZ reporter gene [27] . Western blots Western blots were carried out essentially as previously described [51] using the following primary antibodies (1:1,000 dilution): anti-Nck1/2 (Millipore, Billerica, MA, #06-288), anti-GFP (Covance, Vienna, VA, #MMS-118R), anti-HA (Covance, #MMS-101P), anti-vinculin (Sigma-Aldrich, #V-9131), anti-agarose-myc (BD, #3843-1), anti-myc (Millipore, #05-724), anti-GST (Covance, #MMS-112R). Samples were resolved in 12% SDS–polyacrylamide gels and transferred to PVDF membranes for western blot analysis. Co-immunoprecipitations Co-IPs were carried out essentially as previously described [51] briefly cells were washed with cold PBS and lysed for 10 min at 4 °C. Cell lysates were centrifuged at 14,000 g , and the supernatants were precleared with 15 μl of protein-A-agarose beads (Invitrogen, #15918-014) for 15 min at 4 °C. After a short centrifugation, supernatants were incubated with myc, GFP or Nck antibody (1 μg) or control IgG (at 4 °C for 2 h). Protein-A-agarose beads or anti-mouse-Immunoglobulin G (Sigma, Cat no. A6531) were then added, and mixture was incubated at 4 °C for 1 h. Beads were washed in lysis buffer and boiled. Samples were resolved by immunoblotting standard techniques. Pull-down assays Individual SH3 domains of Nck1 inserted into pGEX-2N (pEBG) were transformed in XL1-blue E. coli cells (Stratagene). Expression and purification of GST fusion Proteins in E. coli were carry out essentially as previously described [52] . COS-1 cells were washed with cold PBS and then lysed in 300 μl of a lysis buffer. Cell lysates were centrifuged at 14,000g, and the supernatants were precleared with 15 μl of gluthatione–Sepharose-beads for 15 min at 4 °C. After a centrifugation, supernatants were incubated with different GST-fused proteins or GST alone (at 4 °C for 2 h). Gluthatione–Sepharose-beads (20 μl) were added, and mixture was incubated at 4 °C for 1 h. Beads were washed in lysis buffer and boiled. Samples were resolved on an SDS–PAGE gel and immunoblotted by standard methods. Surface plasmon resonance SPR measurements were conducted using the Biacore 2000 system, equipped with research grade CM5 sensor chips (Biacore AB, Uppsala, Sweden). Measurements were expressed in arbitrary resonance units. GST-Nck1 SH3 domain was expressed in E. coli and immobilized to the sensor chip using the Amine Coupling kit (GE healthcare). The following peptides biotinylated at the C-terminus were synthesized by GeneScript (Piscataway, NJ): G-QQEAPRPKRIICPREVENRPKYYGRE-L-Biotin (WT-β2-chim), G-QQEAARAKRIICPREVENRPKYYGRE-L-Biotin (AKAKR-β2-chim), G-QQEAPAPAAIICPREVENRPKYYGRE-L-Biotin (PAPAA-β2-chim), G-QQEAPRPKRIICPREVENRAKYYGRE-L-Biotin (P53A-β2-chim). LYQLQQEAPRPKRIICPREVENRPKYYGREFH-L-Biotin (WT-β2-chim long). Association/dissociation cycles were performed at a constant flow rate of 5–10 μl min −1 . Peptides in HBS buffer were injected for 10 min at different concentrations. For dissociation of bound peptides, HBS buffer was injected at a constant flow for 15 min. For chip regeneration, bound peptides were removed by one 30 s pulse injection of 0.1% SDS. Biocore sensorgrams were processed using the BIA evaluation software 3.0. Membrane pelleting assays Expression and purification of the third SH3 domain of Nck1 is described in Supplementary Methods . SLVs containing PMA were prepared according to the method of Mosior et al. [53] . Briefly, PS and lissamine rhodamine-dihexadecanoyl-sn-glycero-3-phosphoethanolamine (Rhodamine-DHPE) were combined in a 65–70:30:0.06 ratio and dried to a thin film. The lipids were resuspended in 20 mM Tris-HCl, pH 7.4, 0.3 M sucrose and vortexed vigorously. PMA (0–5 mol %) was added slowly with vortexing to the resuspended lipid mixture. The lipid mixture was subjected to four freeze-thaw cycles in liquid nitrogen and sonication in a water bath at 25 °C. Three-hundred microlitre of a buffer containing 20 mM Tris, pH 7.4 and 100 mM NaCl were added to 250 μl of the lipid mixture and spun at 100,000 g (30 min, 20 °C), to pellet the SLVs. The SLVs were resuspended in 20 mM Tris, pH 7.4, 150 mM NaCl, 1 mM TCEP to give a final lipid concentration of 1 mM. SLVs containing 0–5 mol % PMA were incubated with 150 pmoles of β2-chimaerin alone to determine the binding constant for PMA binding. Nck1 SH3-3 binding to the same SLVs was determined by incubating 265 pmoles of Nck1 SH3-3. To assay the corecruitment of Nck1 SH3-3 and β2-chimaerin to SLVs containing PMA, 0–3 μmoles of Nck1 SH3-3 in 20 mM Tris, pH 7.4, 150 mM NaCl, 1 mM TCEP were incubated for 30 min at room temperature. The SLV-protein mixture was spun at 100,000 g (30 min at 20 °C) and the supernatant discarded. The pellet was washed with buffer, resuspended and samples of the SLVs containing 50 pmoles of β2-chimaerin were loaded on a 4–12% NuPAGE gel (Invitrogen). β2-chimaerin and/or Nck1 SH3-3 were stained with Coomassie Blue (Safe Stain, Invitrogen) and the bands quantitated at 670 nm (excitation with 633 nm red laser, quantitation with 670 nm BP 30 emission filter) using a Typhoon scanner in fluorescence mode. Binding curves were fitted using a one-site-binding model. FRET studies FRET assays were carried out essentially as described [9] (see also Supplementary Methods ). For YFP photobleaching studies we used a Zeiss LSM710 confocal microscope equipped with an argon laser, and data processed with the ZEN 2011 software. Cells were fixed with 4% paraformaldehyde in PBS (pH 7.4) for 10 min at room temperature. Studies were performed with 40–80 iterations of selected regions of the cell with a 514 nm laser beam. FRET efficiency was calculated from the ratio of the CFP fluorescence observed before (CFPpre) and after (CFPpost) photobleaching, using the following formula: FRET efficiency=1−CFPpre/CFPpost [54] . Modelling analysis The solution structure (NMR) of the SH3-3 domain of human Nck2 (pdb code: 1wx6 ) was used to build a homology model of the Nck1 SH3-3 domain. The template and target sequences were aligned using ClustalW and a 3-D model was generated using MODELLER [55] . MODELLER DOPE (Discrete Optimized Potential Energy) potential function was used to assess the quality of the modelled structures. The overall stereo chemical quality of the models was validated using Ramachandran plot and PROCHECK analysis [56] . The three-dimensional crystal structure of the β2-chimaerin (pdb code: 1wa6 ) and the homology model of Nck1 SH3-3 domains were docked using PyMOL (The PyMOL Molecular Graphics System, Version 1.5.0.1 Schrödinger, LLC) by a two-step process. First, the β2-chimaerin Pro-rich motif was superimposed on the poly-Pro region of the CMS–SH3 heterodimeric complex (pdb code: 2j7i ) by minimizing the root mean square deviation. Subsequently, the Nck1 SH3-3 domain homology model was superimposed on the SH3 domain of the above CMS–SH3 complex using the same algorithm. The resulting docked model was analysed to identify important contacts between Nck1 SH3-3 domain and β2-chimaerin. A similar model of Nck1 SH3-3 interaction with α2-chimaerin was generated by superimposing the crystal structure of the α2-chimaerin on to β2-chimaerin of the previous model. Statistical analysis We used either unpaired Student's t -test or one-way analysis of variance with Bonferroni’s adjustment. How to cite this article: Gutierrez-Uzquiza, A. et al. Coordinated activation of the Rac-GAP β2-chimaerin by an atypical proline-rich domain and diacylglycerol. Nat. Commun. 4:1849 doi: 10.1038/ncomms2834 (2013).